Structural basis of PcsB-mediated cell separation inStreptococcus pneumoniae Separation of daughter cells during bacterial cell division requires splitting of the septal cross wall by peptidoglycan hydrolases. In Streptococcus pneumoniae, PcsB is predicted to perform this operation. Recent evidence shows that PcsB is recruited to the septum by the transmembrane FtsEX complex, and that this complex is required for cell division. However, PcsB lacks detectable catalytic activity in vitro , and while it has been proposed that FtsEX activates PcsB, evidence for this is lacking. Here we demonstrate that PcsB has muralytic activity, and report the crystal structure of full-length PcsB. The protein adopts a dimeric structure in which the V-shaped coiled–coil (CC) domain of each monomer acts as a pair of molecular tweezers locking the catalytic domain of each dimeric partner in an inactive configuration. This suggests that the release of the catalytic domains likely requires an ATP-driven conformational change in the FtsEX complex, conveyed towards the catalytic domains through coordinated movements of the CC domain. In order to divide, bacteria must synthesize a new septal cell wall, which must be split down the middle by one or more murein hydrolases to separate the resulting daughter cells. The precise molecular mechanism underlying this fundamental process is still poorly understood in most bacteria. In the present investigation, we have studied the septal cross wall splitting mechanism in the Gram-positive bacterium Streptococcus pneumoniae . In addition to its important biological implications, this process might be worthy for therapeutic targeting since S. pneumoniae is a major human pathogen that has become increasingly resistant to antibiotics in recent decades [1] . Thus, new drugs and new drug targets are urgently sought. The peptidoglycan (PG), the major constituent of the cell wall, is essential for bacterial survival. Its synthesis and turnover involve a number of enzymes that must function in a coordinated manner. During the last decade it has become clear that a two-component regulatory system termed WalKR (also known as VicKR and YycGF) controls PG metabolism in low G+C Gram-positive bacteria [2] . Analysis of the WalKR regulons of Bacillus subtilis and Staphylococcus aureus have revealed their role in the control of the expression of a number of PG hydrolases, some of which are involved in the separation of daughter cells [3] , [4] . Similarly, genes encoding several putative and proven PG hydrolases are part of the pneumococcal WalKR regulon [5] , [6] . The product of one of these genes, PcsB (from protein required for cell wall separation of group B streptococcus), has been shown to be essential for viability in S. pneumoniae strains D39 and R6 (ref. 7 ). PcsB is a secreted putative murein hydrolase that localizes to the septal area. It has been characterized to various degrees in S. pneumoniae [8] , [9] , Streptococcus mutans (where it is called GbpB) [10] , and Streptococcus agalactiae [11] . In all cases, it has been shown to be required for normal growth and cell division. Homologues of PcsB are present in all members of the genera Streptococcus and Lactococcus . Judging from its primary structure, PcsB consists of four parts: an amino-terminal signal peptide, a coiled–coil (CC) domain containing putative leucine zipper motifs, an alanine-rich linker region and a carboxy-terminal cysteine, histidine-dependent amidohydrolase/peptidase (CHAP) domain. Despite the presence of this putative catalytic domain in the PcsB sequence, attempts to demonstrate hydrolytic activity of full-length PcsB have been unsuccessful [8] , [11] , [12] . Recently, it was discovered that PcsB interacts with the membrane-embedded protein FtsX through its N-terminal CC domain. FtsX has two extracellular loops, ECL1 and ECL2, which are involved in this interaction [13] , [14] . At the cytoplasmic side of the membrane, FtsX, which has four transmembrane segments, interacts with FtsE. An increasing body of knowledge indicates that the FtsEX complex is an essential regulator of murein–hydrolase activity in Gram-positive as well as Gram-negative bacteria [15] . FtsE is an ATPase, and it is therefore believed that ATP hydrolysis drives a conformational change in the FtsEX/PcsB complex that activates PcsB. Recently, PcsB has emerged as a leading candidate for a new-generation pneumococcal vaccine. Depending on the vaccine type, pneumococcal vaccine formulations in the current use contain a mixture of 7–23 capsular polysaccharides, making them costly to produce and with limited serotype coverage. In addition, since there are at least 90 different capsular varieties, serotype replacement and capsular switching will eventually enable pneumococci to evade capsule-based vaccines. A promising alternative is the use of conserved nonpolysaccharide antigens [16] . PcsB, which is a surface-exposed and exceptionally conserved protein (>99.5% identity) among clinical isolates of S. pneumoniae , has demonstrated its efficacy in lethal models of sepsis and pneumonia [17] . In the present report we show that depletion of PcsB in S. pneumoniae strain R6, inhibits daughter cell separation without affecting the synthesis of new septal cross walls. We also provide strong evidence that the C-terminal CHAP domain of PcsB exhibits muralytic activity. Furthermore, the full-length pneumococcal PcsB protein was expressed, purified to homogeneity, crystallized and its structure determined. The structure displays a striking arrangement of the CC and catalytic domains, which associate forming a dimer through three-dimensional domain swapping. In solution, the protein is present in a monomer–dimer equilibrium. Analysis of the structure, together with the biochemical and biophysical characterization, have provided new insights into the catalytic mechanism of PcsB, revealing the regulatory role played by the PcsB–FtsEX complex during daughter cell separation. Effect of PcsB depletion on cross wall separation In Gram-negative bacteria, synthesis and splitting of the new cross wall take place in close succession, leading to a gradual constriction of the whole bacterial cell that culminates in separation. On the other hand, in Gram-positives, it has been reported that the complete cross wall is synthesized before muralytic enzymes cleave it [18] . To determine whether synthesis of the PG cross wall is independent of cross wall splitting, we performed transmission electron microscopy (TEM) studies of PcsB-depleted S. pneumoniae R6 cells. In intermediately depleted R6 cells, the first sign of PcsB deficiency is uncleaved cross walls. As seen in Supplementary Fig. 1 , the original cell wall separating the first-generation daughter cells has not been cleaved, even though the second-generation daughter cells are separated by fully formed cross walls. In severely depleted cells, most new cross walls are misplaced. In these cells, synthesis of the next septum can start anywhere from the internal surface of the cell and, in many cases, it grows at a skewed angle relative to the cell’s long axis. As shown in Supplementary Fig. 1C , a new cross wall can even assemble on top of and at a right angle to an old cross wall. Together, these results show three important facts about PcsB-depleted R6 cells: (i) splitting of PG cross walls are inhibited already in intermediately depleted cells, (ii) the lack of PcsB does not inhibit the synthesis of new cross walls, and (iii) strongly depleted cells lose their spatial orientation and initiates synthesis of new cross walls at random. The last effect may explain why PcsB is essential in the R6 strain. For reasons unknown, some pneumococcal strains are able to survive without PcsB. Deletion of the pcsB gene in these strains gives rise to very sick cells with phenotypes [17] that are highly similar to those depicted in Supplementary Fig. 1 . Overall structure of PcsB The crystal structure of the wild-type PcsB was solved at 2.5 Å resolution by the SAD technique (see Methods). The asymmetric unit of PcsB consists of two monomers arranged in a 164-Å long dimer ( Fig. 1a ). Each monomer is composed of three distinct regions: a CC domain (residues 41–266), a linker region (residues 267–278) and a CHAP domain (residues 279–392) ( Fig. 1b and Supplementary Fig. 2 ). Structures of the two monomers show C α backbone root mean squared deviation (r.m.s.d.) of 1.82 Å; as the domains are nearly identical (C α backbone r.m.s.d. of 1.09 Å and 0.16 Å for CC and CHAP domains, respectively) this value is due to a slight difference in modular arrangement between CC and CHAP domains for each monomer ( Supplementary Fig. 3 ). Thus, hereafter, we limit our discussion to one PcsB molecule (Chain A). The whole structure can be roughly encased in an acute triangle of two long sides (~112 and ~118 Å) and a short side of ~66 Å. The CC domain is arranged in five helices, three long bent helices (α1, α3 and α4) composed of a large number of residues (66, 73 and 41 aa, respectively) and two short ones (α2 and α5). The electron density was of good quality for all of them except for the short α2 that also has the highest B factors. The linker region is composed of an alanine-rich region and the sequence comprises the stretch between Pro271 to Pro278 (266-AAAPVRAKVRP-279). This region connects the end of the α5 helix of the CC domain with the globular catalytic CHAP domain. The electron density for the linker unequivocally defines the connection between the modules of one of the chains ( Supplementary Fig. 4 ), while in the other, the density is of less quality probably due to crystal contacts. The catalytic domain displays an α+β papain-like amidase fold, with two α-helices (α1 c and α2 c ) and an antiparallel β sheet built up by β1 c –β4 c ( Fig. 1b ). The N-terminal lobe (α1 c –α2 c ) folds together with the C-terminal lobe, comprising the β sheet, to build the active-site cleft ( Fig. 1c ). Similar to other amidases, the reactive cysteine of PcsB, Cys292, is positioned at the N-terminal end of α1 c . 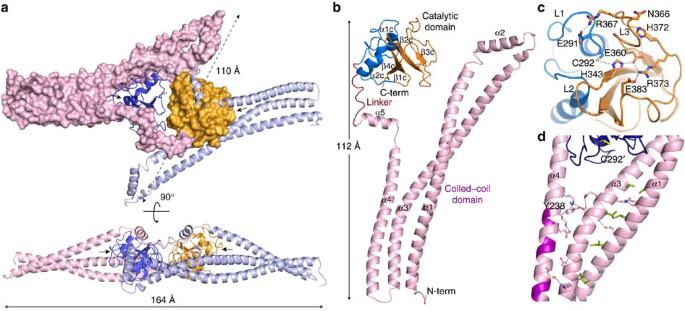Figure 1: Three-dimensional structure of PcsB. (a) Representation of the PcsB dimer showing the molecular surface for monomer A (CC domain coloured in pink and catalytic domain in orange) and the monomer B as a ribbon representation (CC domain coloured in light blue and catalytic domain in dark blue). Arrows indicate the active sites. (b) General structure of PcsB monomer. CC domain (pink) is formed by five helices. An eleven-residue linker region (dark red) connects to the catalytic CHAP domain. The CHAP domain is built by N-lobe (coloured in blue) and C-lobe (coloured in orange), the different secondary structural elements are labelled. (c) Active site of PcsB showing the catalytic residues (Cys292, His343 and Glu360) and the interaction network around the triad. Relevant loops in the active site (L1, L2 and L3) are labelled. The salt bridge interaction (E291-R367) connecting the L1 and L3 loops is also depicted. The previously predicted catalytic Asn366 is far from the active site and oriented outward. (d) Interactions connecting α1, α3 and α4 of the CC domain (pink cartoon). Leu and Ile residues involved in hydrophobic interactions are depicted as green sticks. Residues involved in salt links, and Tyr238, are drawn as pink capped sticks. The Ala-rich regions are coloured in magenta. The CHAP domain of the dimeric partner is represented as blue cartoon and the catalytic Cys292′ as yellow sticks. Figure 1: Three-dimensional structure of PcsB. ( a ) Representation of the PcsB dimer showing the molecular surface for monomer A (CC domain coloured in pink and catalytic domain in orange) and the monomer B as a ribbon representation (CC domain coloured in light blue and catalytic domain in dark blue). Arrows indicate the active sites. ( b ) General structure of PcsB monomer. CC domain (pink) is formed by five helices. An eleven-residue linker region (dark red) connects to the catalytic CHAP domain. The CHAP domain is built by N-lobe (coloured in blue) and C-lobe (coloured in orange), the different secondary structural elements are labelled. ( c ) Active site of PcsB showing the catalytic residues (Cys292, His343 and Glu360) and the interaction network around the triad. Relevant loops in the active site (L1, L2 and L3) are labelled. The salt bridge interaction (E291-R367) connecting the L1 and L3 loops is also depicted. The previously predicted catalytic Asn366 is far from the active site and oriented outward. ( d ) Interactions connecting α1, α3 and α4 of the CC domain (pink cartoon). Leu and Ile residues involved in hydrophobic interactions are depicted as green sticks. Residues involved in salt links, and Tyr238, are drawn as pink capped sticks. The Ala-rich regions are coloured in magenta. The CHAP domain of the dimeric partner is represented as blue cartoon and the catalytic Cys292′ as yellow sticks. Full size image The architecture of the PcsB CC domain The extended CC PcsB is composed of residues arranged in a continuous helical arrangement. Only the first four residues (41–45) and those of the short turns do not follow this pattern. All the helices within the CC domain are located in the same plane except for the α5 helix. The CC domain is a V-shaped molecule formed by helices α1–α3 on one side and by α4 and α5 on the other, making an angle of ~40° ( Fig. 1b ). A search for the closest structural homologues of CC PcsB with the DALI server [19] reveals that no similar structure for the complete CC has been reported previously. High structural homology is, however, found between the antiparallel α1α3 bundle of the CC domain and the human inter-SH2 domains of p85β and p85α, the regulatory subunits of phosphatidylinositol-4,5-biphosphate 3-kinase, the tower domain of the Lys-specific histone demethylase, the molecular chaperone prefoldin and the structures of CC domains from type III secretion system translocators ( Supplementary Fig. 5 ). Remarkably, interhelix interactions in the CC PcsB differ depending on the helices in question: interactions between α1 and α3 are mainly mediated by hydrogen bonds and by the hydrophobic interactions of residues forming a leucine zipper ( Fig. 1d ), in contrast, α3 interacts with α4 through salt links and the hydrophobic contribution is less relevant, as a consequence of the presence of less bulky alanine residues (all the Ala-rich regions, except that of the linker, are located in α4) ( Fig. 1d ). Interestingly, Tyr238 is inserted at the bottom of the V-shaped conformation. Together with long-chain charged residues it opens the cavity in which the catalytic domain of the other paired monomer is located ( Fig. 1d ). The catalytic machinery of the CHAP domain of PcsB A search for proteins structurally related to the catalytic domain of PcsB was performed with the DALI server [19] . Papain-like proteins such as the Staphylococcus saprophyticus CHAP domain protein, the catalytic domain of endolysin PlyCA and the type VI amidase effector Tse1 from Pseudomonas aeruginosa , were found to be among the most closely related 3D structures ( Supplementary Fig. 6a ). Papain-like hydrolytic enzymes form covalent intermediates with their substrates during the course of the reaction. A reactive cysteine acts as a catalytic nucleophile, promoted by the side chain of a histidine. The His-imidazole ring is further hydrogen bonded to a third catalytic residue, usually an Asp or Asn. The Cys-His-Asp/Asn catalytic triad is positioned by the common structural core; the cysteine is located at the N terminus of the helix, and the histidine and the Asp/Asn are provided by the β-sheet and linking loops [20] . Sequence analysis suggested that Cys292, His343 and Asn366 are the catalytic residues in this triad. Mutations in the first two residues (Cys292Ala and His343Ala) are not tolerated in PcsB, whereas that of Asn366Ala is. [7] Our crystal structure indicates that Asn366 is far from the Cys292 ( Fig. 1c ) while the Glu360 is hydrogen bonded to His343 and superimposes with the Asn175 from the catalytic triad of the papain ( Supplementary Fig. 6b ). Therefore, the catalytic triad comprises Cys292, His343 and Glu360 ( Fig. 1c ). The corresponding triad positions are also seen in the secreted CHAP domain from S. saprophyticus [21] and were shown to be the proteolytic triad in pyroglutamyl peptidases, a family of cysteine peptidases [22] . Remarkably, a strong network of salt bridge and hydrogen-bond interactions is observed around the active site of PcsB ( Fig. 1c ). Besides the expected hydrogen bonds between the catalytic triad, Glu360 is making salt bridge interactions with both His372 and Arg373, and the last with Glu383. These interactions could modulate the PcsB activity depending on the protonation state of the corresponding amino acids. Substrate binding in PcsB The active site of PcsB is partially occluded by the presence of the α3 helix from the dimeric partner ( Fig. 1a ), a fact that provides interesting implications for the regulatory role of the CC domain in the PcsB dimer (see discussion below). Among the PG papain amidases, some, as for instance Spr from E. coli, have a closed active-site architecture with active-site loops blocking the active-site entrance. Others like Tse1 from P. aeruginosa present an exposed active site [23] ( Supplementary Fig. 7 ). Similar to Tse1, CHAP PcsB has an open active site with loops L1-L3 ( Fig. 1c and Supplementary Fig. 7 ) protruding outwards, creating a large groove ~31 Å long and ~7 Å wide. The active site of one monomer, chain A, showed an entrapped polyethylene glycol molecule, presumably mimicking binding of the substrate ( Fig. 2a and Supplementary Fig. 8 ). This open active site, however, is partially occluded due to the dimeric arrangement. Very interestingly, the distance between the putative glycan strands is greater than 30 Å (ref. 24 ). Consequently, the active site of PcsB could get access to the peptide bridges that interconnect the glycan strands in the PG sacculus. 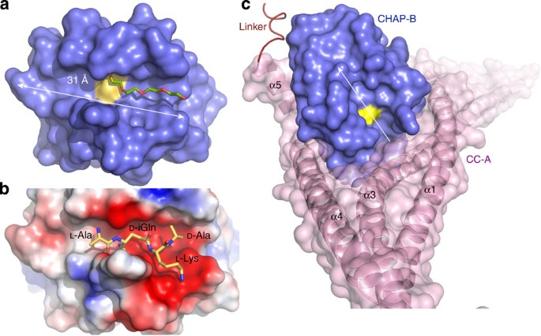Figure 2: The active site of PcsB. (a) Molecular surface representation of the CHAP domain of PcsB. The catalytic Cys292 is coloured in yellow. The PEG molecule attached to the active site is represented as capped sticks. The length of the active-site groove is indicated by an arrow. (b) Electrostatic potential on the CHAPPcsBmolecular surface with the peptideL-Ala-D-isoGln-L-Lys-D-Ala docked in the active site. An acidic patch (coloured in red) stabilizesL-Lys. (c) Domain interactions between the CC domain in chain A (CC-A) with the CHAP domain of chain B (CHAP-B). Colour code as inFig. 1. White arrow indicates, as ina, the active-site groove. Figure 2: The active site of PcsB. ( a ) Molecular surface representation of the CHAP domain of PcsB. The catalytic Cys292 is coloured in yellow. The PEG molecule attached to the active site is represented as capped sticks. The length of the active-site groove is indicated by an arrow. ( b ) Electrostatic potential on the CHAP PcsB molecular surface with the peptide L -Ala- D -isoGln- L -Lys- D -Ala docked in the active site. An acidic patch (coloured in red) stabilizes L -Lys. ( c ) Domain interactions between the CC domain in chain A (CC-A) with the CHAP domain of chain B (CHAP-B). Colour code as in Fig. 1 . White arrow indicates, as in a , the active-site groove. Full size image All attempts to obtain crystals of a complex between PcsB and PG analogues failed, very likely due to the occlusion created by the dimer arrangement. To gain insight into the substrate recognition by PcsB, we performed docking calculations with GOLD [25] using a peptide stem fragment, L -Ala- D -isoGln- L -Lys- D -Ala, present in pneumococcal PG. The top scoring positions nicely fit the polyethylene glycol molecule found at the active site of the crystal structure ( Fig. 2a,b ) and place the scissile bond between isoGln and L -Lys close to the catalytic Cys292 and His343. The ligand is strongly stabilized by many hydrogen bonds and salt links with residues in the active site ( Supplementary Fig. 9 ). Remarkably, a very similar conformation for the substrate ( L -Ala-D-Glu-mDAP) was found in Tse1 from P. aeruginosa [23] where mDAP is present in place of L -Lys. It has been shown that Tse1 exhibits a strong preference for the mDAP-type [23] . Our docking calculations reveal the presence of an acidic patch in the PcsB active site formed by Asp338 and Glu383 ( Fig. 2b and Supplementary Fig. 9 ), responsible of stabilization of L -Lys in the cross-linked PG. This patch does not exist in Tse1, and consequently provides an explanation for the different substrate specificities of the two PG amidases. CHAP PcsB displays murein–hydrolase activity To investigate whether full-length PcsB has muralytic activity, we performed zymography with purified recombinant PcsB and pneumococcal cells mixed into the separating SDS–PAGE gel as substrate. Consistent with the results reported by others [8] , [11] , [12] , no muralytic activity was detected. Next, we expressed only the C-terminal CHAP domain of PcsB. For purification purposes, a 6xHis tag was attached to the N-terminal end of the domain (see Methods). Zymography analysis performed with various amounts of the CHAP PcsB protein revealed distinct clearing zones in the opaque gel at the expected migration positions ( Fig. 3a,b ). As a negative control, we expressed a mutated version of the CHAP domain (His-CHAP C292A ) in which the catalytic cysteine was substituted with an alanine. No clearing zones were observed when the same amounts of the CHAP PcsB(C292A) -mutant protein was subjected to zymography ( Fig. 3a,b ). Together, these results provide strong evidence that the catalytic domain has muralytic activity and further support the open conformation observed in the crystal structure of CHAP PcsB . In order to identify the exact bond split by PcsB, purified PG was treated with CHAP PcsB in solution. Subsequent analysis of the digest by reverse phase HPLC, however, did not reveal any cleavage products. Thus, it remains for future studies to determine the cleavage specificity of PcsB. 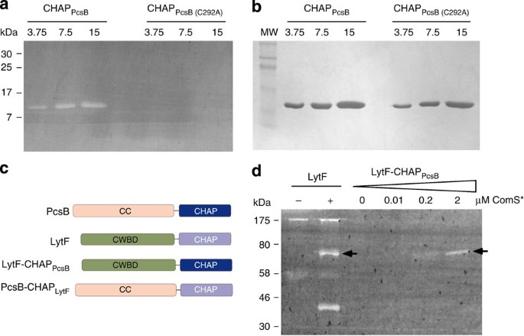Figure 3: Zymogram analysis demonstrating the PG–hydrolyzing activity of His-CHAPPcsBand the LytF-CHAPPcsBchimera. (a) Muralytic activity of His-CHAPPcsB.Different amounts of purified His-CHAPPcsBand its C292A-mutated counterpart (3.75, 7.5 and 15 μg indicated on top) were separated in an SDS–PAGE gel containing RH14 cells as substrate. The light bands are clearing zones showing degradation of the PG of the RH14 cells incorporated in the SDS–PAGE gel. (b) A parallel gel without RH14 cells was stained with Coomassie Blue to visualize the purified His-CHAPPcsBand His-CHAPPcsB(C292A)recombinant proteins loaded onto the gel ina. (c) Cartoon depicting the domain composition of PcsB and LytF, and the chimera (LytF-CHAPPcsBand PcsB-CHAPLytF) constructed by swapping the domains of the parental proteins. The LytF-CHAPPcsBchimera was used in the zymogram analysis displayed below ind. The gene encoding the PcsB-CHAPLytFchimera was incorporated into the genome ofS. pneumoniaestrain R6 to determine whether the chimeric protein was able to replace the essential PcsB wild-type protein (see result section for details). (d) Zymogram analysis. Lanes: MW, molecular weight marker; LytF (−), extracts ofS. gordoniicells; LytF (+), extracts of competence inducedS. gordoniicells producing LytF; LytF-CHAPPcsB(0–2), extracts of pneumococci expressing increasing amounts of LytF-CHAPPcsBchimera from the ComS*-inducible PComXpromoter30. ComS* is an 8 aa synthetic peptide that is added to the growth medium to induce transcription of genes inserted behind the PComXpromoter. Maximum expression is reached at 2 μM ComS* (see text for details). The light bands in lanes containing cell extracts are clearing zones that result from degradation of the PG sacculus ofS. gordoniicells that have been incorporated in the SDS–PAGE separating gel. Left arrow: clearing zone corresponding to wild-type LytF. Right arrow: clearing zone corresponding to the LytF-CHAPPcsBchimera. Figure 3: Zymogram analysis demonstrating the PG–hydrolyzing activity of His-CHAP PcsB and the LytF-CHAP PcsB chimera. ( a ) Muralytic activity of His-CHAP PcsB. Different amounts of purified His-CHAP PcsB and its C292A-mutated counterpart (3.75, 7.5 and 15 μg indicated on top) were separated in an SDS–PAGE gel containing RH14 cells as substrate. The light bands are clearing zones showing degradation of the PG of the RH14 cells incorporated in the SDS–PAGE gel. ( b ) A parallel gel without RH14 cells was stained with Coomassie Blue to visualize the purified His-CHAP PcsB and His-CHAP PcsB(C292A) recombinant proteins loaded onto the gel in a . ( c ) Cartoon depicting the domain composition of PcsB and LytF, and the chimera (LytF-CHAP PcsB and PcsB-CHAP LytF ) constructed by swapping the domains of the parental proteins. The LytF-CHAP PcsB chimera was used in the zymogram analysis displayed below in d . The gene encoding the PcsB-CHAP LytF chimera was incorporated into the genome of S. pneumoniae strain R6 to determine whether the chimeric protein was able to replace the essential PcsB wild-type protein (see result section for details). ( d ) Zymogram analysis. Lanes: MW, molecular weight marker; LytF (−), extracts of S. gordonii cells; LytF (+), extracts of competence induced S. gordonii cells producing LytF; LytF-CHAP PcsB (0–2), extracts of pneumococci expressing increasing amounts of LytF-CHAP PcsB chimera from the ComS*-inducible P ComX promoter [30] . ComS* is an 8 aa synthetic peptide that is added to the growth medium to induce transcription of genes inserted behind the P ComX promoter. Maximum expression is reached at 2 μM ComS* (see text for details). The light bands in lanes containing cell extracts are clearing zones that result from degradation of the PG sacculus of S. gordonii cells that have been incorporated in the SDS–PAGE separating gel. Left arrow: clearing zone corresponding to wild-type LytF. Right arrow: clearing zone corresponding to the LytF-CHAP PcsB chimera. Full size image Modular arrangement and oligomerization in PcsB A dimeric arrangement of PcsB molecules was found in the crystal structure ( Fig. 1a ). This dimer is formed by three-dimensional domain swapping [26] , in which both monomers exchange their catalytic domains in a similar way to that originally described for the dimeric structure of diphtheria toxin [27] . The dimer places both catalytic domains in the middle with their active sites oriented in opposite directions, and with the CC domain extending outwards on the same axis in a 164 Å long dimer. Analysis of the PcsB dimer by the PISA server [28] , gave a high value for the complex formation significance score (0.915) and indicated that the buried area upon assembly formation is 7,040 Å 2 . The calculated free energy of assembly dissociation (Δ G diss ) is 26.1 kcal M −1 . The Δ G diss corresponds to the free energy difference between dissociated and associated states. Positive values of Δ G diss indicate that an external driving force should be applied in order to dissociate the assembly. Consequently, the PcsB assembly is predicted to be thermodynamically stable. The V-shaped CC domain of one monomer clamps the CHAP domain of the other in a narrow cavity. All the α helices of the CC domain, except for the α2 helix, are involved in the interaction with the CHAP domain. While there are few hydrogen bonds and no salt links between the two domains ( Supplementary Table 1 ), about three-quarters of the CC/CHAP interactions are van der Waals contacts, most of which involve exposed hydrophobic side chains ( Supplementary Fig. 10 and Supplementary Table 1 ). In agreement with crystallographic results, analytical ultracentrifugation experiments over a broad range of protein concentrations (0.1–8.0 mg ml −1 ) revealed that the protein exists as an equilibrium mixture of dimers and monomers in solution, with dimer favored at higher protein concentrations (over 4 mg ml −1 ) and monomer at low concentrations ( Supplementary Fig. 11 ). The monomer–dimer equilibrium presents an estimated K d of 90 μM. Interestingly, while the experimental sedimentation coefficients for the dimer are compatible with that calculated for the crystallographic dimeric structure, those for the monomer are better described by a PcsB molecule with the CHAP domain inserted in its own CC domain rather than the protein monomer observed in the asymmetric unit of our crystal ( Supplementary Fig. 11 ). We explored whether the arrangement in the crystal is representative of PcsB in solution using small-angle X-ray scattering (SAXS). The overall molecular parameters derived from the scattering data are given in Supplementary Table 2 . The scattering profiles at five different concentrations (0.29–9.40 mg ml −1 ) ( Fig. 4 and Supplementary Fig. 12 ) indicate the presence of a monomer–dimer equilibrium, being the monomer more abundant at lower concentrations whereas the dimer is the predominant form at higher concentrations. A molecular mass of 61±6 kDa was deduced for the dimer, which is comparable with the expected dimer mass of 78 kDa ( Supplementary Table 2 ). The radius of gyration ( R g ) and the maximum dimension ( D max ) with values of 45±3 Å and 168±7 Å, respectively, indicate a rather extended dimeric assembly in agreement with the dimensions observed in the crystal structure ( D max of 164 Å, see Fig. 1a ). The ab initio models generated with DAMMIF and DAMMIN without symmetry constrains produced rather elongated shapes of PcsB at high concentration. Rigid-body modelling was performed using the dimer found in the crystal structure, showing that the envelope encases the main core of the dimer ( Fig. 4c ). It is worth to note that the α2 regions that present the highest B factors in the crystal structure are not observed in the SAXS envelope of the dimer. At low concentrations (0.29–1.18 mg ml −1 ) PcsB appeared mostly as a monomer with a molecular mass and R g between 35±4/44±4 kDa and 35±6/41±6 Å, respectively ( Supplementary Table 2 ). The D max for monomers ( Supplementary Table 2 ) were also compatible with their associated crystallographic monomer (122 Å). Rigid-body modelling of the PcsB monomer extracted from the crystallographic dimer inside the SAXS envelope, fits well the elongated CC domain (coloured in orange in Fig. 4b ) but not the linker or the CHAP domain (coloured in blue in Fig. 4b ) indicating that a single-molecular conformation alone does not represent the experimental data fittingly. Remarkably, if the catalytic domain is replaced with the one corresponding to its dimeric partner (coloured in red in Fig. 4b ) the model perfectly fits the SAXS envelope. Therefore, two relevant points can be derived from this analysis; first, in solution, the monomeric PcsB present an inactive conformation with the CHAP domain inserted in its own CC domain, and second, the PcsB dimer is generated by the three-dimensional domain swapping of their catalytic domains. 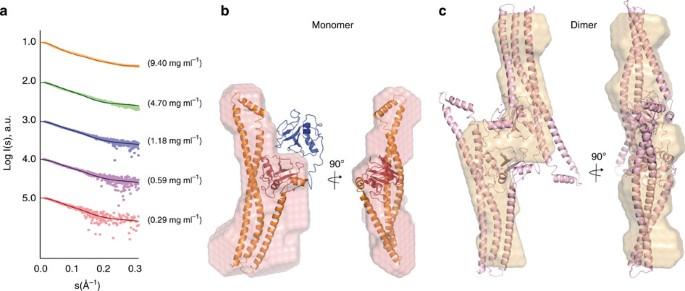Figure 4: Arrangement of PcsB in solution by SAXS. (a) SAXS experimental scattering curves (dots) and theoretical scattering computed from the models (smooth curves) at different concentrations of PcsB. The data for different concentrations were offset vertically for clarity. a.u., arbitrary units. (b) Rigid-body overlaying of theab initiodetermined SAXS envelope and the PcsB crystallographic monomer. The elongated CC domain (coloured in orange) fits into the envelope but not the linker or the CHAP domain (coloured in blue). In red, a model where the catalytic domain belongs to the dimeric partner, that perfectly fits the SAXS envelope. (c) Rigid-body fitting of the PcsB crystallographic dimer inside the SAXS envelope. The region around the α2 helix presents the highest B factors in the crystal structure, and is not observed in the SAXS envelope of the dimer. Figure 4: Arrangement of PcsB in solution by SAXS. ( a ) SAXS experimental scattering curves (dots) and theoretical scattering computed from the models (smooth curves) at different concentrations of PcsB. The data for different concentrations were offset vertically for clarity. a.u., arbitrary units. ( b ) Rigid-body overlaying of the ab initio determined SAXS envelope and the PcsB crystallographic monomer. The elongated CC domain (coloured in orange) fits into the envelope but not the linker or the CHAP domain (coloured in blue). In red, a model where the catalytic domain belongs to the dimeric partner, that perfectly fits the SAXS envelope. ( c ) Rigid-body fitting of the PcsB crystallographic dimer inside the SAXS envelope. The region around the α2 helix presents the highest B factors in the crystal structure, and is not observed in the SAXS envelope of the dimer. Full size image Evidence that PcsB muralytic activity is regulated by its modular arrangement We have previously characterized a murein hydrolase termed LytF [29] , which is produced by Streptococcus gordonii strain Challis during the competent state. LytF consists of an N-terminal cell wall binding domain and a C-terminal CHAP domain. The C-terminal CHAP domains of PcsB and LytF are the same size and 70% identical, while their N-terminal domains are unrelated. Considering that CHAP PcsB and CHAP LytF are highly similar ( Supplementary Fig. 13 ), we wondered whether CHAP PcsB would become active if fused to the N-terminal domain of LytF. To test this idea, we replaced the CHAP domain of LytF with the CHAP domain of PcsB. The resulting LytF-CHAP PcsB chimera was expressed in pneumococcal cells from the ComS*-inducible P comX promoter [30] . Extracts from pneumococcal cultures grown in the presence of 0, 0.01, 0.2 and 2 μM ComS* were subjected to zymography with S. gordonii cells incorporated in the separating gel ( Fig. 3c,d ). The analysis revealed a clearing zone corresponding to the expected molecular weight of LytF-CHAP PcsB in the sample induced with 2 μM ComS*. The fact that the LytF-CHAP PcsB chimera gives rise to clearing zones in gels containing S. gordonii cells as substrate shows that the structure and composition of the peptide cross bridges of S. pneumoniae and S. gordonii must be similar. Available data indicate that the pentapeptide stem L -Ala- D -isoGln- L -Lys- D -Ala- D -Ala is the same in the two species. In S. pneumoniae interpeptide bridges are either absent or predominantly L -Lys- L -Ser- L -Ala- D -Ala, while they are predominantly L -Lys- L -Ala- L -Ala- D -Ala in S. gordonii [31] , [32] . To further verify that the function of PcsB depends on the muralytic activity of its CHAP domain, we constructed a chimera in which the CHAP domain of PcsB was replaced by the corresponding domain of LytF. LytF, which is produced by S. gordonii cells during the competent state, lyses susceptible streptococcal cells by disrupting their cell wall [29] . The gene encoding this PcsB-CHAP LytF chimera was inserted into the native pcsB locus in a strain that expressed the wild-type PcsB ectopically from the P comX promoter. Next, the wild-type gene was deleted from the ectopic locus giving rise to strain SPH250. Surprisingly, the SPH250 strain was viable. A homology model for the PcsB-CHAP LytF chimera was constructed ( Supplementary Fig. 13 ). This model indicates that the main determinants for catalytic activity and substrate recognition were conserved between both CHAP domains. Despite some of the interactions stabilizing CC and CHAP domains in PcsB (such as a poly-Ala region) could be disturbed in the chimera ( Supplementary Fig. 13 ) the strain SPH250 is viable. Its doubling time of 45 min was somewhat longer than the 35 min generation time of the parental strain. In addition, inspection of the SPH250 cultures by light microscopy revealed some enlarged misshapen cells, morphological changes reminiscent of those seen in pneumococcal cells that have been subjected to light PcsB depletion ( Supplementary Fig. 14 ). Together, these results provide strong evidence that the CHAP domain of PcsB has muralytic activity that is regulated by the CC domain. The crystal structure of the PG amidase PcsB reveals a surprising arrangement of its different domains. The CC domain is a unique V-shaped molecule built by three long bent α-helices and two short ones. A flexible and extended 11-aa linker connects the CC domain with the catalytic CHAP domain. Remarkably, the crystal structure of the full-length PcsB is a dimer formed by three-dimensional domain swapping in which the entire catalytic domain of one monomer is inserted in the internal cavity of the CC domain of the other ( Figs 1a and 2c ), a pattern that is also observed for the monomer in solution as deduced from AUC and SAXS experiments. The PISA server further confirmed the stability of this dimer formation, as well as by analytical ultracentrifugation and by SAXS experiments. In this unique oligomeric arrangement, the CC domain of one monomer acts as molecular tweezers clamping the catalytic domain of its dimeric partner. The implications of this arrangement are profound; active sites are partially occluded (roughly half of the active-site groove) by the α3 helix of the partner resulting in an inactive dimer. This point was confirmed by our experiments with the CHAP PcsB domain and a LytF-CHAP PcsB chimera in which the CHAP LytF domain of the LytF fratricine was replaced by the closely related CHAP PcsB domain of PcsB. When separated from the CC domain, the CHAP PcsB domain turned out to be active on its own in zymography assays. Similarly, when fused to the cell wall binding domain of LytF, the CHAP domain of PcsB displayed muralytic activity ( Fig. 3 ). In contrast, muralytic activity was not observed with the full-length PcsB protein. The functional homology of the CHAP PcsB and CHAP LytF domains was demonstrated by showing that replacement of PcsB in strain R6 with a chimera consisting of the CC domain of PcsB and the CHAP domain of LytF gave rise to viable R6 cells. The role of the CC domain, however, goes beyond its inhibitory function. The structural framework provided by the CC domain is also required for activation of PcsB, that is, for cross wall splitting and daughter cell separation. It has been reported that a temperature sensitive (Ts) mutant containing two amino-acid changes (L79S and L218P, R6 strain numbering) in the CC domain of PcsB showed mild or severe defects in cell morphology and division at 32 °C or 41.4 °C, respectively [13] . At the non-permissive temperature, the double mutant formed spherical cells that phenocopied the defect caused by severe depletion of PcsB [13] . The three-dimensional structure of PcsB shows that these mutations are located in the leucine zipper regions and are involved in the interaction between α1 and α3 (Leu 79) and in the interaction between α4 and α3 (Leu218) ( Supplementary Fig. 15 ). Thus, the alteration in the CC architecture caused by these amino-acid changes probably perturbs the activation mechanism of PcsB and locks the mutant protein in an inactive state, although we cannot discard other possibilities such as the mutant is unstable and degraded, or that mutations in the CC domain could alter the length of the protein or its orientation relative to the cytoplasmic membrane. The conserved FtsEX complex recently emerged as a major regulator of PG hydrolysis during bacterial cell division [13] , [15] , [33] . FtsEX is essential or conditionally essential in a great variety of bacterial species [14] , [34] . FtsEX structurally resembles an ABC transporter [35] , but recent studies indicate that FtsEX acts as a signal transduction system rather than as a transporter of an unknown substrate [34] . The 3D structure of PcsB provides clues to how regulation/activation by the FtsEX complex can take place ( Fig. 5 ). The dimeric arrangement of PcsB precludes any lytic activity unless the CHAP domain is released, in a controlled way, from the CC domain. To release the CHAP domain, the ‘molecular tweezers’, which consists of α1–α3 on one side and α4–α5 on the other, must be opened on both sides. Previous studies involving Ts and suppressor mutants of PcsB and FtsX, respectively, revealed mutations in the large (ECL1) and small (ECL2) extracellular loops of FtsX that indicate that the FtsX–PcsB interaction occurs between these loops and the CC domain of PcsB [13] , [14] . The Ts mutations in CC PcsB are located just in the middle of α1 and α3 helices and at the base of α4 helix ( Supplementary Fig. 15 ), while the connecting regions in FtsX involve the distal portion of the ECL1 and ECL2 loops [14] . These results point to a specific interaction between the FtsX loops and both sides of the ‘molecular tweezers’. The energy required for the coordinated movement of α-helices in the CC PcsB domain is in all likelihood produced by hydrolysis of ATP by FtsE. In agreement with this, it has been shown that the conserved amino acids in the ATP binding site of FtsE are essential for pneumococcal growth, supporting the idea that ATPase activity by FtsE is required for FtsEX→PcsB signalling and coordination of cell separation [14] . Once released, the catalytic domain would not require further opening of the active-site loops. We have demonstrated that CHAP alone exhibits hydrolytic activity and presents a pre-formed 31-Å groove that can accommodate the cross-linked peptide stems ( Fig. 5c ). Our docking calculations allowed us to map the different subsites of substrate-peptide recognition for PcsB. Especially relevant is the presence of an acidic patch that could explain PcsB’s specificity for L -Lys containing stem peptides ( Fig. 2b and Supplementary Fig. 9 ). Further studies on hydrolytic activity of PcsB are, however, required to precisely identify the cleavage site of this enzyme. 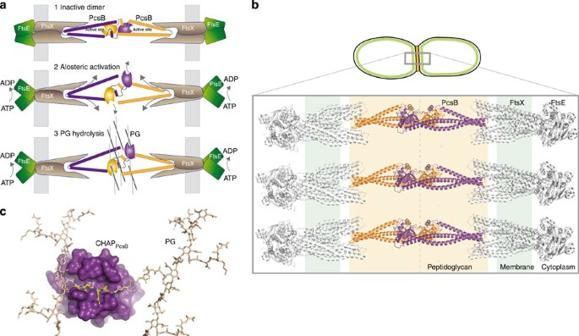Figure 5: Activation and regulation in PcsB. (a) Proposed model for regulation of hydrolytic activity of PcsB. The inactive dimer is located at the septum by FtsX (1). The ATPase activity of FtsE induces an allosteric change on PcsB through FtsX producing the release of the CHAP domains (2). The catalytic domains start the PG hydrolysis (3). (b) Possible spatial location of PcsB dimers (yellow and magenta ribbon) on the pneumococcal septum. The structure of the FtsEX complex resembles that of an ABC transporter (PDB code 2ONJ, is coloured in white ribbons representing FtsEX). (c) Model of the cross-linked PG chains (capped sticks) bound at the molecular surface of the CHAPPcsB(magenta). The peptide substrate used in docking calculations is highlighted (with C atoms in yellow, N atoms in blue and O atoms in red). Figure 5: Activation and regulation in PcsB. ( a ) Proposed model for regulation of hydrolytic activity of PcsB. The inactive dimer is located at the septum by FtsX (1). The ATPase activity of FtsE induces an allosteric change on PcsB through FtsX producing the release of the CHAP domains (2). The catalytic domains start the PG hydrolysis (3). ( b ) Possible spatial location of PcsB dimers (yellow and magenta ribbon) on the pneumococcal septum. The structure of the FtsEX complex resembles that of an ABC transporter (PDB code 2ONJ, is coloured in white ribbons representing FtsEX). ( c ) Model of the cross-linked PG chains (capped sticks) bound at the molecular surface of the CHAP PcsB (magenta). The peptide substrate used in docking calculations is highlighted (with C atoms in yellow, N atoms in blue and O atoms in red). Full size image Our TEM studies of intermediately and severely PcsB-depleted cells show that the synthesis of new cross walls continues unimpeded in the absence of PcsB, suggesting that the cross wall splitting machinery operates independently of the septal PG synthesis machinery. What controls the activity of the cross wall splitting machinery to ensure that it acts at the right time and place? As discussed above, evidence strongly supports that ATP hydrolysis by FtsE provides the energy needed to activate PcsB. However, as ATP is abundant in the cytoplasm throughout the cell cycle, the availability of this nucleotide cannot be a factor that controls splitting of the cross wall. In principle, the level of PcsB, FtsX, FtsE or possibly other hitherto unknown members of the cell wall splitting machinery could be tightly regulated in a cell cycle dependent manner, but so far no evidence of such regulation has been reported. In our view, the unusual dimeric structure of PcsB is a striking characteristic that must serve a critical function in the in vivo regulation of this murein hydrolase. A pertinent question is: Why is the dimer linear with CHAP domains in the middle and CC domains at each end? An intriguing possibility is that dimers form in vivo when a monomer (in the inactive configuration observed in the analytical ultracentrifugation and SAXS experiments) from each of the daughter cells meet in the middle of the cross wall. As shown in Fig. 5 , this implies that the PcsB dimer extends across the cross wall and interacts with FtsEX complexes at both ends. Measurements from TEM micrographs showed that the thickness of the pneumococcal cross wall is in the range of 17–25 nm. It is reasonable to assume that the periplasmic part of FtsX will add a few nanometres to each end of the 16.4 nm long PcsB dimer. Consequently, the estimated thickness of the cross wall is consistent with the model depicted in Fig. 5b . The appealing feature of this model is that splitting of the shared cross wall involves active participation of both daughter cells. Presumably, this introduces an additional level of control in the division process. If PcsB can only function as a dimer, it means that it can only be active in cleaving cross walls and not ordinary cell walls. Only cross walls have membranes on both sides that make it possible to insert PcsB from the compartment of each daughter cell so that the molecules will meet in the middle and dimerize. This would represent an ingenious control mechanism. Due to the net-like polymeric structure of PG, the mobility of PcsB dimers is probably restricted. Thus, it is likely that PcsB, which is a moderately abundant protein in the pneumococcal cell (about ~5,000 monomers per cell [12] ), only acts locally and is then discarded. This is supported by the fact that relatively large amounts of PcsB are released to the medium during growth [12] . In sum, our results indicate that the unique modular structure and dimeric organization of PcsB have evolved to allow precise splitting of the septum during cell division, while avoiding damage to other parts of the PG sacculus. Bacterial growth and transformation Strains of Escherichia coli were grown in Luria Bertani medium at 37 or 28 °C with shaking in the presence of 100 μg ml −1 ampicillin when appropriate. E. coli was transformed by heat shock as described by Sambrook and Russell [36] . S. pneumoniae strain R6 and S. gordonii strain Challis were grown without shaking at 37 °C in C medium [37] and Todd–Hewitt medium (Difco), respectively. Construction of S. pneumoniae mutants was performed by natural transformation. Briefly, pneumococcal cultures were cultivated at 37 °C until they reached OD 550 =0.05–0.1. Then, transforming DNA and 250 ng ml −1 of synthetic competence stimulating peptide were added. After further incubation at 37 °C for 120 min, transformants were selected on Todd–Hewitt plates containing the appropriate antibiotic; kanamycin (400 μg ml −1 ) or streptomycin (200 μg ml −1 ). Expression and purification of mature PcsB PcsB was purified by using the tandem affinity tag called CHiC-tag as previously described by Stamsås et al. [38] followed by ion exchange chromatography. In brief, pcsB fused to the CHiC-tag by overlap extension PCR [39] was cloned into the expression vector pRSET A (Invitrogen) resulting in pGS01 (ref. 38 ). E. coli BL21 (DE3) (Invitrogen) containing the plasmid pGS01 (strain gs32, see Supplementary Table 3 ) was grown at 37 °C with shaking. When reaching OD 600 =0.3 expression of CHiC-fused PcsB was induced by adding isopropyl-β- D -thiogalactopyranoside (IPTG) to a final concentration of 0.1 mM. After incubation for 4 h at 28 °C cells from 2 l of cell culture were harvested at 5,000 g and resuspended in 40 ml 10 mM Tris-HCl (pH 7.4) containing 100 mM NaCl. The cells were lysed by adding lysozyme to a final concentration of 1 mg ml −1 . CHiC-PcsB was purified from the soluble protein fraction by DEAE-cellulose affinity chromatography as described by Sanchez-Puelles et al. [40] The CHiC-tag was then separated from PcsB by digestion with AcTEV Protease (Invitrogen) at 30 °C for 3 h. The free CHiC-tag, undigested CHiC-PcsB and AcTEV Protease, all of which contains a 6xHis tag, were removed by Ni(2+)-NTA affinity chromatography. The flow through which contained PcsB in 10 mM Tris-HCl (pH 7.4) was then bound onto an anion exchanger (Sepharose Q, GE Healthcare) and eluted by gradually increasing the NaCl concentration from 0–500 mM in a 25 ml gradient. The flow rate was set to 1 ml min −1 . The fractions containing >99% pure PcsB were pooled and concentrated by using Amicon Ultra-15 Centrifugal Filter Units (Millipore). Cloning and production of SeMet-PcsB A SeMet derivative of PcsB was produced in order to solve the phase problem associated with the structure determination of native PcsB. Since mature PcsB only contains two methionines per 365 residues (M140 and M150), we introduced two additional methionines by replacing the residues Q180 and L250 with M. Methionine codons were introduced at codon 180 and 250 by overlap extension PCR [39] . For the CAA180 to ATG180 (Q180M) substitution, base pairs 535–1179 of pcsB were amplified using the forward primer ds85 and the T7 reverse primer producing PCR product 1 (Primers are listed in Supplementary Table 4 ). The region corresponding to base pairs 1–559 of pcsB fused 5′ to the CHiC-tag was amplified using the T7 forward primer and reverse primer ds86 producing PCR product 2. The plasmid pGS01 (ref. 38 ) served as template in both reactions. Since primer ds85 is complementary to primer ds86, PCR product 1 and 2 were fused in an overlap extension PCR by using the flanking primers T7 forward and T7 reverse generating PCR product 3. To introduce the additional CTT250 to ATG250 (L250M) substitution, base pairs 748–1179 of pcsB were amplified using forward primer ds79 and T7 reverse primer producing PCR product 4. Similarly region 1–773 of pcsB fused 5′ to the CHiC-tag was amplified using the T7 forward primer and reverse primer ds80 to generate PCR product 5. PCR product 3 was used as template in both reactions. PCR fragment 4 and 5 were fused in an overlap extension PCR using the T7 forward and T7 reverse primers. This generated PCR fragment 6 that contained a Q180M and L250M version of PcsB fused N-terminally to the CHiC-tag. This mutated version of PcsB will be referred to as PcsB mut . Fragment 6 was cleaved with Xba I and Eco RI and ligated immediately downstream of the T7lac promoter in pRSET A giving rise to plasmid pGS214. For production of SeMet-PcsB mut , E. coli BL21 (DE3) harbouring pGS214 (strain ds122, see Supplementary Table 3 ) was grown in M9 minimal medium containing 0.4% glucose [36] and 50 mM choline chloride. Choline was supplemented to M9 to improve the solubility of CHiC-PcsB mut . At OD 600 =0.3 methionine production in E. coli BL21 (DE3) was blocked by adding the following cocktail of amino acids: L -lysine (0.1 mg ml −1 ), L -phenylalanine (0.1 mg ml −1 ), L -threonine (0.1 mg ml −1 ), L -isoleucine (0.05 mg ml −1 ), L -leucine (0.05 mg ml −1 ) and L -valine (0.05 mg ml −1 ). After 10 min, the production of selenomethionine-derivatized CHiC-PcsBmut was induced by adding a final concentration of 0.1 mM IPTG and 0.05 mg selenomethionine (Acros Organics) per ml growth medium. The cells were grown at 28 °C for 4 h before SeMet-derivatized CHiC-PcsB mut was purified as described above for native PcsB. Construction of His-CHAP and pcsB/lytF chimeras To construct the pcsB-CHAP lytF chimeric gene, pneumococcal pcsB without its CHAP-encoding part (bp 1–858) was amplified using the primer pair 216/52 and genomic DNA from strain RH1 (ref. 41 ) as template. The CHAP-encoding part of lytF (bp 1260–1578) was amplified using the primer pair 53/217 and genomic DNA from S. gordonii (Challis) as template. These two fragments were fused by overlap extension PCR using the primer pair 216/217 producing the fragment pcsB-CHAP lytF . Next, ~1,000-bp fragments corresponding to the 5′ and 3′ flanking regions of pcsB were amplified with the primer pairs 37/218 and 219/38, respectively. Genomic DNA from the RH1 strain was used as template. By overlap extension PCR the 5′ flanking region was fused to the 5′ end of the pcsB-CHAP lytF gene using the primer pair 37/217. Similarly, the 3′ flanking region was fused to the 3′ end of pcsB-CHAP lytF using the primer pair 216/38. Finally, these two fragments were fused using the primers 37 and 38. To test if PcsB-CHAP lytF could substitute for wild-type PcsB in S. pneumoniae we wanted to replace the native pcsB gene with the chimeric pcsB-CHAP lytF gene. As pcsB is an essential gene in S. pneumoniae R6, an extra copy of the wild-type gene had to be expressed ectopically before the native pcsB gene could be removed and replaced by a Janus cassette [42] . For ectopic expression of pcsB , we employed the R6 derivative SPH131, which has the ComRS expression/depletion system integrated in its genome [30] . First, the pcsB gene was amplified with the primers 35 and 36 and DNA from strain RH1 as template. Next, fragments corresponding to the ~1,000-bp upstream and downstream regions of the Janus cassette in strain SPH131 were amplified using the primer pairs khb31/khb36 and khb33/khb34, respectively. Then, by the use of overlap extension PCR with the primers khb31 and 36, the pcsB fragment was fused to the upstream fragment. Similarly, the pcsB fragment was fused to the downstream fragment by using the primers 35 and khb34. Finally, these two fragments were fused using the primer pair khb31/khb34. By replacing the Janus cassette in SPH131 with the resulting PCR product strain SPH246 was generated. Before the pcsB-CHAP lytF gene could be introduced into the native pcsB locus, the native pcsB gene was replaced with the Janus cassette. The Janus cassette was amplified with the primers Kan484.F and RpsL41.R and genomic DNA from strain RH426 [32] as template. Fragments (~1,000 bp) corresponding to the 5′ and 3′ regions of the native pcsB gene was amplified using the primer pairs 37/39 and 40/38, respectively. DNA from strain RH1 was used as template. The resulting fragments were then fused to the Janus cassette in separate PCR reactions. The 5′ flanking region was fused to the Janus cassette using the primers 37 and RpsL41.R, while the 3′ flanking region was fused to the Janus cassette with the primers Kan484.F and 38. Finally, these two fragments were fused together using the primers 37 and 38. By transforming strain SPH246 with a PCR fragment corresponding to the Janus cassette flanked by the upstream and downstream regions of the pcsB gene, strain SPH247 was obtained. Transformants of SPH247 was grown in the presence 1 μM ComS* to drive ectopic expression of PcsB. Next, the Janus cassette in SPH247 was replaced with the pcsB-CHAP lytF fragment described above, giving rise to strain SPH248. For removal of the ectopically expressed copy of WT pcsB in strain SPH248, this gene and its P comX promoter was replaced by a Janus cassette. Genomic DNA from strain SPH154 (ref. 43 ), which contains a Janus cassette inserted in the ectopic locus, served as template to amplify a PCR fragment consisting of the Janus cassette plus ~1,000 bp flanking regions. The PCR reaction was carried out with the primers khb31 and khb34. The resulting fragment was transformed into strain SPH248, generating strain SPH249. Finally, the Janus cassette was removed by transforming strain SPH249 with a fragment containing only the flanking regions of the Janus cassette. The 5′ and the 3′ region of the Janus cassette were amplified using the primer pairs khb31/khb32 and 154/khb34, respectively. DNA from SPH154 served as template. These two fragments were fused by overlap extension PCR using the primer pair khb31/khb34. The resulting fragment was transformed into strain SPH249, giving rise to strain SPH250. To construct lytF-CHAP pcsB , the region (bp 76–1332) encoding the cell wall binding domain of LytF (without its 25 aa leader sequence) was amplified using the primer pair ds95/ds96 and DNA from S. gordonii strain Challis as template. The CHAP-encoding region of PcsB (bp 859–1179) was amplified using the primer pair ds97/ds98 and DNA from S. pneumoniae RH1 as template. These two fragments were fused in an overlap extension PCR with the flanking primers ds95 and ds98 resulting in a lytF-CHAP pcsB chimera. LytF-CHAP PcsB was expressed in S. pneumoniae by using the ComRS system described by Berg et al. [30] The 5′ and 3′ regions of the Janus cassette in strain SPH131 (see above) were amplified by the primer pairs khb31/khb36 and khb33/khb34, respectively, and then fused to the 5′ and 3′ ends of the lytF-CHAP pcsB fragment by overlap extension PCR using the primers khb31 and khb34. The resulting fragment was transformed into strain SPH131, replacing the Janus cassette and giving rise to strain SPH252. To construct His-CHAP PcsB , we amplified the CHAP-encoding part of pcsB using the primers ds147 and T7 reverse primer and the plasmid pGS01 (ref. 38 ) as template. The C292A-mutated version of CHAP PcsB was amplified using the same primers but with genomic DNA from SPH258 as template. Primer ds147 contains a 6xHis encoding part. The PCR products were cleaved with Xba I and Eco RI and ligated into pRSET A immediately downstream of the T7lac promoter. The resulting plasmids were transformed into E. coli BL21 (DE3) giving rise to strain ds179 and ds189. Zymogram analysis The muralytic activity of LytF-CHAP PcsB , His-CHAP PcsB and His-CHAP PcsB(C292A) was examined in zymogram gels. For LytF-CHAP PcsB strain SPH252 was grown in the presence of 0, 0.01, 0.2 and 2 μM ComS* inducer for 1 h to drive LytF-CHAP PcsB expression. Competence induced S. gordonii (Challis) was used as control for native LytF activity [29] . The cells were collected at OD 550 =0.25 by centrifugation and lysed in SDS sample buffer. Total protein extracts were separated by SDS–PAGE using a 12% separation gel containing S. gordonii (Challis) cells as substrate. The cell substrate was collected from a 300 ml S. gordonii (Challis) culture at OD 550 =0.3. The cells were suspended in 1.25 ml separation gel buffer (1.5 M Tris–HCl, pH 8.8) and heat inactivated at 95 °C for 10 min before they were mixed into the resolving gel. After gel electrophoresis the gel was washed two times for 30 min in distilled water before protein refolding was initiated by submerging the gels in 50 mM NaCl, 20 mM MgCl 2 , 0.5% Triton X-100 and 20 mM Tris–HCl, pH 7.4. The gels were incubated in refolding buffer until muralytic activity was observed as clear bands in the opaque gel. Similarly, the activity of His-CHAP PcsB and its C292A-mutated counterpart were examined in zymogram gels containing S. pneumoniae strain RH14 as substrate. His-CHAP PcsB and His-CHAP PcsB(C292A) were expressed in E. coli strain ds179 and ds189, respectively by adding a final concentration of 0.1 mM IPTG at OD 600 =0.3 followed by incubation at 28 °C for 4 h. A volume of 500 ml-induced ds179 cells were collected by centrifugation at 5,000 g for 5 min. The cells were then resuspended in 5 ml of 10 mM Tris–HCl, pH 7.4 containing 100 mM NaCl. The cells were lysed by adding lysozyme to a final concentration of 1 mg ml −1 followed by 10 min at 37 °C. His-CHAP PcsB and His-CHAP PcsB(C292A) were purified from the soluble protein fraction by using Protino Ni-TED150 (Macherey–Nagel) columns as described by the manufacturer. The purified proteins were then separated by SDS–PAGE in 13% zymogram gels before the gels were incubated in refolding buffer. Transmission electron microscopy SPH247 cells were grown to an OD 550 =0.3 in the presence of 1 μM ComS*, harvested by centrifugation and washed once in C medium to remove excess ComS*. To start depletion of pcsB , the washed cells were resuspended in C medium containing 0 μM ComS* to an OD 550 =0.025. Cells were collected for TEM 1 h before their growth rate was affected by PcsB starvation and 45 min after the cell growth was severely inhibited by pcsB depletion. Cells were fixed by mixing cell culture and fix solution (2% paraformaldehyde [v/v] and 2.5% glutardialdehyde [w/v] in 0.1 M sodium cacodylate buffer pH 7.4) in a 1:1 ratio. After incubation at room temperature for 1 h, the cells were fixed overnight at 4 °C. The fixed cells were washed three times in sodium cacodylate buffer (0.1 M, pH 7.4). For TEM, fixed cells were post fixed for 1 h at room temperature using 1% OsO 4 (w/v) and 1.5% K 3 [Fe(CN) 6 ] (w/v) dissolved in dH 2 O. Following three washing steps in dH 2 O (3 × 10 min), cells were prestained for 30 min using 1% uranyl acetate. Next, cells were washed for 3 × 10 min in water, and dehydrated with a gradient series of ethanol comprising 10 min sequential incubations in 70, 90 and 100% ethanol. Finally, the cells were stepwise infiltrated in LR white resin as follows: LR white resin: EtOH in ratios 1:3 for 30 min, 1:1 overnight, 3:1 for 4 h and finally 100% LR white resin overnight followed by embedding in 100% LR white resin at 60 °C overnight. Thin sections were cut with a diamond knife mounted on an ultramicrotome (LEICA, EM UC 6). The sections were counterstained with 1% KMnO 4 for 10 min. After staining, the grids were washed thoroughly in dH 2 O. The sections were examined in a FEI MORGAGNI 268 electron microscope. PcsB crystallization Crystals of native PcsB were obtained using the sitting-drop vapour diffusion method at 4 °C. Crystals grew in 2 μl droplets formed by mixing 1 μl of protein solution at 10 mg ml −1 (buffered in 20 mM Tris-HCl pH 7.5) and 1 μl of precipitant solution formed by 12% (v/v) polyethylenglycol 4000, 0.1 M Hepes pH 7.5, 0.2 M Magnesium Acetate in 1:1 volume ratio drops supplemented with 115,38 mM Guanidinium chloride and 33.5 mM n-octyl-β- D -Glucopyranoside. Crystals belong to the P3 1 21 hexagonal space group ( a = b =125.8 Å, c =126.6 Å). PcsB SeMet derivative crystals were obtained in the same way as the native PcsB crystals but replacing magnesium acetate by zinc acetate in the reservoir solution. SeMet derivative crystals belong to the P3 1 21 hexagonal space group ( a = b =127.2 Å, c =126.3 Å). X-ray data collection and structural determination Crystals were harvested in a proper reservoir solution supplemented with 23% ethylene glycol, mounted into nylon loops and flash cooled in liquid nitrogen. Native and SAD experiments were carried out on beamline ID29 at the European Synchrotron Radiation Facility (ESRF) (Grenoble, France). All X-ray data sets were processed and scaled with XDS [44] and Aimless [45] , respectively. PcsB structure was solved by SAD technique. Due to the low content of methionine residues (2 Met residues) in the wt PcsB sequence, four different constructions were produced having two additional methionine residues. Among them only the PcsB-Q180M-L250M construct could be expressed in the presence of SeMet, purified and crystallized. PcsB-Q180M-L250M crystals diffracted up to at 2.71 Å resolution. The initial selenium sites were located with SHELX [46] using the HKL2MAP GUI [47] and refined within AUTOSHARP [48] . Solvent flattening was calculated with Parrot [49] followed by density modification with Pirate programme [50] . Initial model was obtained with Buccaneer [51] followed by manual modelling with COOT [52] . Two monomers were found in the asymmetric unit yielding a Matthews’s coefficient of 3.97 Å 3 /Da and a solvent content of 69.07%. All X-ray data sets presented anisotropy, the best of the native PcsB being collected at 2.55 Å resolution. The PcsB-SeMet derivative structure was used as initial model in the molecular replacement method using Phaser [53] . Structure of native PcsB was subjected to alternate cycles of refinement with Refmac5 [54] and COOT. Geometry of the final models was checked with MOLPROBITY [55] . In all cases, the good quality of all electron density maps allowed modelling the most part of the polypeptide chain, ligands and solvent molecules (see Table 1 ). The first 40 amino acids from the N-terminal tail were disordered and were not visible in the structure and the short helix α2 presented a poor electron density especially in one of the monomers. In the crystal structure of the native PcsB, the electron density map clearly defines a polyethylene glycol moiety attached to the active site of chain B. The figures were generated by using PyMol (Molecular Graphics System, Version 1.5.0.4 Schrödinger, LLC.). Table 1 Diffraction data collection and refinement statistics. Full size table Docking calculations The structure of the pneumococcal PG peptide stem fragment L -Ala- D -isoGln- L -Lys- D -Ala was modelled using PyMol. Charges assignment and optimization were carried in chimera [56] . Molecular docking was carried using GOLD (Genetic Optimization for Ligand Docking) software [25] , using the genetic algorithm (GA). The PEG ligand found in the crystal structure was used as starting point for cavity detection. For each of the 25 independent GA runs, a maximum number of 100,000 GA operations were performed on a set of five groups with a population size of 100 individuals. Default cut-off values of 2.5 Å (dH-X) for hydrogen bonds and 4.0 Å for van der Waals distance were employed. When the top three solutions attained r.m.s.d. values within 1.5 Å, GA docking was terminated. The r.m.s.d. values for the docking calculations are based on the r.m.s.d. matrix of the ranked solutions. Best-ranked solutions were always among the first 10 GA runs, and the conformation of molecules based on the best fitness score was further analysed. Analytical ultracentrifugation Sedimentation velocity was used in combination with sedimentation equilibrium to determine the association state of protein PcsB over a broad range of concentrations (0.1–8.0 mg ml −1 ). Sedimentation velocity runs were carried out at 171,600 g and 20 °C in an XL-I analytical ultracentrifuge (Beckman–Coulter) equipped with ultraviolet-Vis and Raleigh interference detection system, using an An50Ti rotor and 3 and 12 mm double sector centerpieces (sample in the range of 0.1–1.0 mg ml −1 were loaded in normal 12 mm centrepiece and samples in the range of 2.0–8.0 mg ml −1 in narrow 3 mm centerpieces). The sedimentation coefficient distributions were calculated by least squares boundary modelling of sedimentation velocity data using the c ( s ) method [57] as implemented in the SEDFIT programme. Calculated s- values were corrected to standard conditions (water, 20 °C, and infinite dilution) using the SEDNTERP programme [58] and the concentration dependence of s , to get the corresponding standard s- values. Short column (21–85 μl, depending of the centerpieces) equilibrium runs were carried out at multiple speeds (5,426 g, 11,394 g and 17,804 g) and the corresponding scans were measured at the appropriate wavelength. Whole cell apparent weight-average buoyant molecular weight of the protein samples were determined by fitting a single-species model to the experimental data using the HeteroAnalysis programme [59] . The corresponding protein molecular weights were calculated from the experimental buoyant values using 0.722 cm 3 g −1 as the protein partial specific volume. Several models of self-association were globally fitted to multiple sedimentation equilibrium using the HeteroAnalysis programme. To assign the most probable structure of the main protein species present, the standard s- values experimentally obtained were compared with the s -values determined for given structural models using the shell model calculation implemented in HYDROPRO [60] . SAXS experiments SAXS data were collected at the EMBL beamline BM29 at the ESRF (Grenoble, France), using a robotic sample changer, from six sample solutions of PcsB at concentrations ranging from 0.29–9.40 mg ml −1 in 10 mM Tris-HCl pH 7.4 and 5% glycerol at 277 K. Data were recorded using a photon-counting Pilatus 1 M pixel detector (DECTRIS, Switzerland) at a sample detector distance of 2.7 m and a wavelength of λ =1 Å. The scattering intensity I(q) was recorded in a range of the momentum transfer 0.01< q <0.6 Å −1 (where q =4 π sin θ / λ , and 2 θ is the scattering angle). Sample solutions were circulated in a thermostatic flow mode during the measurement to minimize radiation damage effects. Ten frames of 1-s exposures were collected for each sample, normalized to the transmitted intensity and subsequently averaged using AUTOSUB. In PRIMUS, the forward scattering I(0) and the radii of gyration Rg were estimated using the Guinier approximation I ( q )= I (0) exp(−( qR g) 2 /3) with qR g<1.3. These parameters were also computed from the entire scattering patterns using the indirect transform package GNOM, providing also the pair-distance distribution function P(r) , from which the maximum particle dimension, Dmax , was estimated. The molecular weight was calculated from excluded volume of the hydrated particle (the Porod volume, V p). The ab initio modelling programs DAMMIN and DAMMIF were used for low-resolution shape generation, and 10 models were calculated in the slow mode, and averaged with DAMAVER, which also provides a value of normalized spatial discrepancy representing a measure of similarity among different models. The theoretical profile from the high-resolution structure of PcsB was computed with CRYSOL. The ab initio model was superimposed with the high-resolution structure using the programme SUPCOMB. All the SAXS programs and calculation modules are included in the ATSAS programs package [61] . Accession codes : Atomic coordinates and structure factors for native PcsB have been deposited in the Protein Data Bank with accession code 4CGK . How to cite this article : Bartual, S. G. et al. Structural basis of PcsB-mediated cell separation in Streptococcus pneumoniae . Nat. Commun. 5:3842 doi: 10.1038/ncomms4842 (2014).